Re-examining extreme carbon isotope fractionation in the coccolithophoreOchrosphaera neapolitana 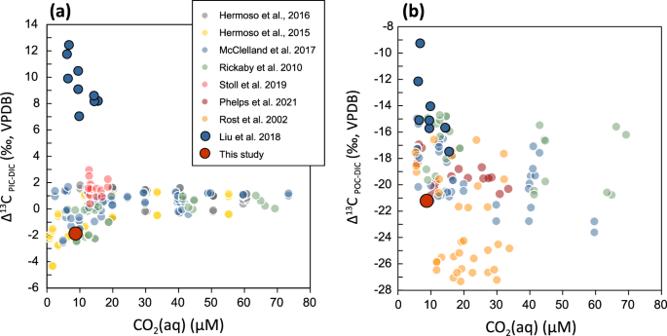Fig. 1: Carbon isotope fractionations (Δ13C) of coccolithophores in different laboratory culture studies. aCarbon isotope fractionation between PIC (particulate inorganic carbon from harvested cells) and DIC (dissolved inorganic carbon from seawater).bCarbon isotope fractionation between POC (particulate organic carbon from harvested cells) and DIC. Markers plotted in red and blue areOchrosphaera neapolitanain this study and in Liu et al.1, respectively. Markers in other colors are results from other publications2,3,4,12,13,14,15using different species of coccolithophores includingCoccolithus pelagicus,Gephyrocapsa oceanica,Calcidiscus leptoporus, andEmiliania huxleyi. 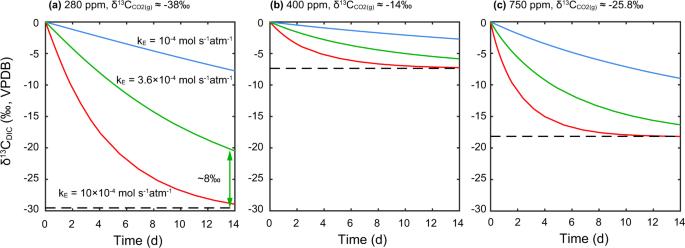Fig. 2: Simulated DIC carbon isotope ratios evolution during bubbling. Panel a, b, c are simulations for differentpCO2 and initial δ13CDIC. Blue curves:kE= 10−4mol s−1atm−1(a slower equilibrium). Red curves:kE= 10−3mol s−1atm−1(a faster equilibrium). Green curves:kE= 3.6 × 10−4mol s−1atm−1(potential exchanging rate for Liu et al.1). The black dashed lines represent the isotopic equilibrium δ13CDIC. The disequilibrium between DIC and gas in 280 ppm treatment after two weeks of bubbling is marked by the vertical green arrows. Laboratory culture Ochrosphaera neapolitana (RCC1357) was precultured in K/2 medium without Tris buffer [8] using artificial seawater (ASW) supplemented with NaHCO 3 and HCl to yield an initial DIC of 2050 µM. In triplicate, 1-L bottles were filled with 150 mL of seawater medium with air in the bottle headspace and inoculated with a mid-log phase preculture at an initial cell concentration of 10 4 cells mL −1 . Cultures were grown at 18 °C under a warm white LED light at 100 ± 20 µE on a 16h-light/8h-dark cycle. Bottles were orbitally shaken at 60 rpm to keep cells in suspension. Cell growth was monitored with a Multisizer 4e particle counter and sizer (Beckman Coulter). At ~1.4 × 10 5 cells mL −1 , cells were diluted up to 300 mL to 2–3 × 10 4 cells mL −1 and harvested after 2 days of more exponential growth up to 7.9 ± 0.6 × 10 4 cells mL −1 . More detailed culture results are listed in the Supplementary Note 1 . Immediately after harvesting, pH was measured using a pH probe calibrated with Mettler Toledo NBS standards (it should be noted here that high ionic strength calibration standards would be optimal for pH measurement of liquids like seawater). There was a carbonate system shift during the batch culture and more details are shown in Supplementary Fig. S1 . Cells in 50 mL were pelleted by centrifuging at ~1650 × g for 5 min. Seawater supernatant was analyzed for DIC and δ 13 C DIC by injecting 3.5 mL into an Apollo analyzer and injecting 1 mL into He-flushed glass vials containing H 3 PO 4 for the Gas Bench. For seawater DIC, an Apollo SciTech DIC-C13 Analyzer coupled to a Picarro CO 2 analyzer was calibrated with in-house NaHCO 3 standards dissolved in deionized water at different known concentrations and δ 13 C values from −4.66 to −7.94‰. δ 13 C DIC in media were measured with a Gas Bench II with an autosampler (CTC Analytics AG, Switzerland) coupled to ConFlow IV Interface and a Delta V Plus mass spectrometer (Thermo Fischer Scientific). Pelleted cells were snap-frozen with N 2 (l) and stored at −80 °C. For PIC analysis, pellet was resuspended in 1 mL methanol and vortexed. After centrifugation, the methanol phase with extracted organics was removed and the pellet containing the coccoliths was dried at 60 °C overnight. About 300 mg of dried coccolith powder were placed in air-tight glass vials, flushed with He and reacted with five drops of phosphoric acid at 70 °C. PIC δ 13 C and δ 18 O were measured by the same Gas Bench system. The system and abovementioned in-house standards were calibrated using international standards NBS 18 (δ 13 C = −5.01‰, δ 18 O = +23.00‰) and NBS 19 (δ 13 C = +1.95‰, δ 18 O = +2.2‰). The analytical error for DIC concentration and δ 13 C is <10 μM and 0.1‰, respectively. POC and PON were determined from cells harvested on pre-combusted QFF filters and deep-frozen until analysis. Inorganic carbon from cells on filters was removed by fuming sulfurous acid during 24 h. Filters were placed inside a desiccator on a porous tray and 50 mL sulfurous acid below was fumed with a vacuum pump. Gases were evacuated and filters were further dried at 60 °C overnight. Right before Elemental Analysis (EA), filters were compacted and wrapped into tin cups with the help of tweezers and a press. Samples loaded on a 96-well plate were combusted in the oxidation column at 1020 °C of a Thermo Fisher Flash-EA 1112 coupled with a Conflo IV interface to a Thermo Fisher Delta V-IRMS (isotope ratio mass spectrometer). Combustion gas passed through a reduction column at 650 °C producing N 2 and CO 2 which were separated by chromatography and into a split to the IRMS for an on-line isotope measurement. Simulations of carbon isotope evolution during aeration The DIC carbon isotope evolution model is simplified from the model in Zhang et al. [7] The exchanging rate (with a unit of mol s −1 ) between CO 2 (g) and CO 2 (aq) depends on the CO 2 gradient and exchanging rate constant ( k E , with a unit of ppm s −1 ): ER = k E (CO 2( g ) – k H CO 2(aq) ), where the k H is Henry’s law constant with a unit of ppm µM −1 . The evolutions of DIC and DIC carbon isotope ratios during CO 2 aeration can be calculated by four differential equations: 
    dC/dt= k_E/V(G-C k_H)+(k_-1H^++k_-4)C-(k_+1+k_+4 OH^-) B  XB1
 (1) 
    d^13C/dt=k_E/V( ^13G α_g2aq- ^13C k_Hα_aq2g)+(k_+1^13+k_+4^13OH^-) ^13B X^13B1-(k_-1^13 H^++k_-4^13) ^13C
 (2) 
    dB/dt=- (k_-1H^++k_-4 )C+(k_+1+ k_+4 OH^-) B  XB1
 (3) 
    d^13B/dt=-(k_-1^13H^++k_-4^13) ^13C+(k_+1^13+k_+4^13 OH^-) ^13B  X^13B1
 (4) where capital letters G, C, B, H, and OH represent CO 2 (g), CO 2 (aq), HCO 3 − + CO 3 2− , H + , and OH − , respectively. The V stands for volume. The α is the isotopic fractionation, e.g. α g2aq represents the carbon isotope fractionation of CO 2 gas diffusion into liquid phase. The XB1 and X 13 B1 are the fraction of HCO 3 − in (HCO 3 − + CO 3 2− ) and the fraction of H 13 CO 3 − in (H 13 CO 3 − + 13 CO 3 2− ). The XB1 can be calculated by \({{{{{\rm{XB}}}}}}1=\frac{1}{1+\frac{K2}{\left[{{{{{{\mathrm{H}}}}}}}^{+}\right]}}\) and the X 13 B1 can be calculated by \({{{{{{\rm{X}}}}}}}^{13}{{{{{\mathrm{B}}}}}}1=\frac{1}{1+\frac{K2}{\left[{{{{{{\mathrm{H}}}}}}}^{+}\right]}{\alpha }_{{{{{{{\mathrm{CO}}}}}}_{3}}-{{{{{{\mathrm{HCO}}}}}}_{3}}}}\) , where the \({\alpha }_{{{{{{{\mathrm{CO}}}}}}}3-{{{{{{\mathrm{HCO}}}}}}}3}\) is the carbon isotope fractionation between CO 3 2− and HCO 3 − [9] . The k +1 is the reaction rate constant of CO 2 hydration, which can be calculated by \({{{{{\rm{ln}}}}}}{k}_{\!+1}=1246.98-\,\frac{61900}{{T}_{k}}-183{{{{{\rm{ln}}}}}}{T}_{k}\) [10] . The k −1 , the reaction rate constant of HCO 3 − dehydration, can be calculated from k +1 , \({k}_{-1}=\,\frac{{k}_{+1}}{K1}\) . The k −4 and k +4 are the reaction rate constants of CO 2 hydroxylation and HCO 3 − dihydroxylation. The k +4 is calculated by \(\,{{{{{\rm{ln}}}}}}{k}_{+4}=17.67- \,\frac{2790.47}{{T}_{k}}\) [10] and \({k}_{-4}={k}_{+4}\frac{{K}_{{{{{{\mathrm{w}}}}}}}}{K1}\) , where K w is the stoichiometric ion product of water. The K 1 and K 2 are the first and second dissociation constants of carbonic acid and in this study, we employed equations from [11] , in which the K1 and K2 were calculated for pH in NBS scale. The reaction rate constants for 13 C ( \({k}_{-1}^{13}\) , \({k}_{+1}^{13}\) , \({k}_{-4}^{13}\) and \({k}_{+4}^{13}\) ). The initial values for these differential equations are described in the Supplementary Note 2 .